Bacterial effector modulation of host E3 ligase activity suppresses PAMP-triggered immunity in rice Pathogen effector proteins are delivered to host cells to suppress plant immunity. However, the mechanisms by which effector proteins function are largely unknown. Here we show that expression of XopP Xoo , an effector of rice pathogen Xanthomonas oryzae pv. oryzae , in rice strongly suppresses peptidoglycan (PGN)- and chitin-triggered immunity and resistance to X. oryzae . XopP Xoo targets OsPUB44, a rice ubiquitin E3 ligase with a unique U-box domain. We find that XopP Xoo directly interacts with the OsPUB44 U-box domain and inhibits ligase activity. Two amino-acid residues specific for the OsPUB44 U-box domain are identified, which are responsible for the interaction with XopP Xoo . Silencing of OsPUB44 suppresses PGN- and chitin-triggered immunity and X. oryzae resistance, indicating that OsPUB44 positively regulates immune responses. Thus, it is likely that XopP Xoo suppresses immune responses by directly interacting with and inhibiting a positive regulator of plant immunity. Immunity in plants is generally initiated with the recognition of the pathogen- or microbe-associated molecular patterns (PAMPs/MAMPs), including bacterial flagellin or peptidoglycan (PGN), and fungal chitin [1] , [2] , [3] , [4] . The recognition of PAMPs by pattern-recognition receptors (PRRs) triggers PAMP-triggered immunity (PTI). PTI constitutes the first layer of plant immunity that restricts pathogen proliferation. To interfere with host PTI, plant pathogens secrete a variety of effector proteins into host cells, allowing the pathogen to manipulate host physiology to promote pathogen growth [5] . Some of the effectors interact either directly or indirectly with the intracellular immune receptors of the nucleotide-binding leucine-rich repeats, triggering a second layer of immune responses often accompanied with hypersensitive cell death, which is referred to as effector-triggered immunity (ETI) [1] . Ubiquitination is an important post-translational modification in eukaryotic cells and is involved in a variety of plant processes, such as hormone signalling, immunity, flowering, cell cycle, circadian rhythm control, growth and development [6] . The ubiquitination process involves sequential enzymatic activities. Ubiquitin is activated by a ubiquitin-activating enzyme (E1). The activated ubiquitin is then transferred to a ubiquitin-conjugating enzyme (E2). Ubiquitin ligase (E3) mediates ubiquitin transfer from an E2 to a target protein. Eukaryotic E3 ligases are classified into two major classes, RING (really interesting new gene) finger/U-box and HECT (homologous to E6-associated protein C-terminus), according to the mechanism of ubiquitin transfer [6] . RING finger/U-box proteins transfer ubiquitin directly from the E2 to the target proteins, whereas HECT proteins form thioester intermediates with ubiquitin before ligating it to the target. The U-box and RING finger domains are structurally similar, although the U-box lacks the characteristic zinc-chelating cysteine and histidine residues [7] . Recent studies revealed that RING finger/U-box ubiquitin ligases are implicated in many aspects of plant immune responses [8] . Tobacco U-box E3 ubiquitin ligase CMPG1 regulates programmed cell death in ETI [9] . Arabidopsis AtPUB22, AtPUB23 and AtPUB24, closely related to CMPG1, negatively regulate immune reactions in response to multiple PAMPs [10] . More recently, AtPUB12 and AtPUB13 were shown to ubiquitinate FLS2, an Arabidopsis receptor for bacterial flagellin (flg22, a conserved 22-amino-acid (aa) peptide from flagellin), resulting in the attenuation of immune signalling by degradation of FLS2 (ref. 11 ). AtPUB17 is implicated in ETI mediated by two nucleotide-binding leucine-rich repeats RPM1 and RPS4 (ref. 12 ). A rice U-box protein SPL11, the closest homologue of AtPUB12 and AtPUB13, is a negative regulator of plant cell death [13] . Rice RING finger protein APIP6 positively regulates resistance to Magnaporthe oryzae [14] . Together, the accumulating evidence indicates that plant U-box (PUB)/RING finger proteins play central roles in plant immune responses. Recently, these U-box/RING finger proteins were reported to be targeted by pathogen effectors. CMPG1 and APIP6 are targeted by Phytophthora infestans effector AVR3a and M. oryzae effector AvrPiz-t, respectively [14] , [15] , [16] . Nevertheless, the molecular mechanisms describing how the effectors inhibit these E3 ligases remain to be identified. Xanthomonas oryzae pv. oryzae ( Xoo ) causes bacterial blight of rice, one of the most important rice diseases in much of Asia [17] . Xoo uses the type III secretion system to secrete the effectors into rice cells. Furutani et al. [18] identified 16 effectors in Xoo . Among them, XopY Xoo (Xoo1488) was shown to strongly suppress host PTI in rice [19] . Recently, we reported that XopY Xoo targets OsRLCK185, a rice receptor-like cytoplasmic kinase that interacts with OsCERK1, a PRR for chitin and PGN [19] . In response to PAMP recognition, OsCERK1 directly phosphorylates OsRLCK185 to transmit the immune signals. The OsCERK1-mediated phosphorylation of OsRLCK185 is suppressed by XopY Xoo , resulting in the inhibition of immune responses including MAP kinase activation [19] , [20] . Expression of the Xoo effector XopAA Xoo (Xoo2875) in rice cells also inhibits PTI [21] . XopAA Xoo targets OsBAK1, a co-receptor for many PRRs, and OsBRI1, a brassinosteroid receptor, as supported by the observation that transgenic plants expressing XopAA Xoo exhibit a brassinosteroid-insensitive phenotype [21] . In addition, XopN, XopR and XopX also have been shown to suppress host immune responses in plants [22] , [23] , [24] . The type III effectors from other Xanthomonas genera have been well documented to suppress host immune responses. AvrAC suppresses FLS2-mediated immune responses by transferring uridyl to BIK1, a RLCK family kinase and an essential immediate signalling partner of FLS2 (ref. 25 ). XopD represses host ethylene responses by desumoylating SIERF4, a tomato transcription factor [26] . XopD also targets Arabidopsis transcription factor MYB30 (ref. 27 ). XopN interacts with a tomato atypical receptor-like kinase and TFT1 (ref. 28 ). XopJ interacts with the proteasomal subunit RPT6 to inhibit proteasome activity [29] . Thus, these recent investigations have revealed that the effectors target key components controlling host immune responses in plants. Therefore, it is likely that identifying the host targets for the effectors will facilitate a more complete molecular understanding of how pathogens inhibit host immune responses. In this study, we found that XopP Xoo , one of the Xoo effectors, suppresses host resistance to Xoo , and PGN- and chitin-induced immune responses, and identified a U-box-type E3 ubiquitin ligase, OsPUB44, as an interacting protein with XopP Xoo . Silencing of OsPUB44 reduces PGN- and chitin-induced immunity and resistance to Xoo , suggesting that OsPUB44 positively regulates immune responses in rice. XopP Xoo interactes with the U-box domain of OsPUB44; however, XopP Xoo is not able to interact with other PUB proteins closely related to OsPUB44. The limited interaction between XopP Xoo and OsPUB44 is dependent on two amino-acid residues specific for the U-box domain of OsPUB44. The interaction of the U-box domain with XopP Xoo results in suppression of the OsPUB44 ubiquitin ligase activity. These results indicate that XopP Xoo modulates the OsPUB44 ligase activity by direct association with the U-box domain for Xoo virulence in rice. XopP Xoo suppresses the PTI response in rice XopP Xoo (Xoo3222), a X. oryzae pv. oryzae type III effector, belongs to a XopP family that is conserved in Xanthomonads [18] ; however, the biochemical functions of the XopP family have not yet been identified. In fact, members of the XopP family do not contain any functional domains predicted from their amino-acid sequences. To investigate how XopP Xoo functions in rice cells, we generated six independent transgenic rice lines expressing XopP Xoo ( XopP Xoo -OX), and two of them were used for pathological experiments. The expression of XopP Xoo mRNAs in rice plants was confirmed by semi-quantitative reverse transcription (RT)–PCR ( Supplementary Fig. 1 ). The XopP Xoo -OX plants did not exhibit any morphological phenotypes ( Supplementary Fig. 2 ). We inoculated the XopP Xoo -OX lines with the T3SS-deficient hrpX mutant of Xoo that is incapable of type III effector delivery [18] , [19] . Because inoculation of the Xoo hrpX mutant induces a strong PTI response in rice, the Xoo hrpX mutant did not cause any disease lesions in wild-type (non-transformed) plants ( Fig. 1a,b ). In contrast, the XopP Xoo -OX plants had severe disease lesions following infection with the Xoo hrpX mutant. Bacterial populations of the Xoo hrpX mutant in the XopP Xoo -OX leaves were significantly higher than in wild-type plants ( Fig. 1c ). In addition, we examined the resistance of XopP Xoo -OX plants to wild-type Xoo by using Xoo T7174R, a spontaneous rifampicin-resistant mutant derived from the wild-type isolate Xoo MAFF311018. The XopP Xoo -OX plants developed larger disease lesions than the wild type ( Fig. 1d,e ), and bacterial growth in the XopP Xoo -OX plants was also slightly higher than the growth in the wild type ( Fig. 1f ). Thus, XopP Xoo likely inhibited immunity induced by infection with both Xoo strains. Although the XopP Xoo -knockout Xoo strain was generated and inoculated on wild-type rice plants, the strain had no defects in virulence ( Supplementary Fig. 3 ). 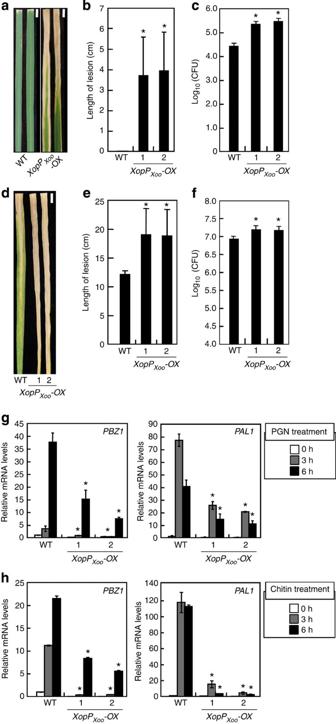Figure 1: XopPXoosuppresses host immune responses. (a) Transgenic plants expressing XopPXoowere more susceptible to theXoo hrpXmutant. Disease lesions were photographed at 25 d.p.i. Scale bar, 10 mm. (b) The lesions induced by infection with theXoo hrpXmutant were measured at 25 d.p.i. (c) The size of theXoo hrpXmutant population in two independentXopPXoo-OX transgenic lines was determined at 5 d.p.i. CFU, colony-forming unit. (d) Transgenic plants expressing XopPXoowere more susceptible toXooT7174R, a spontaneous rifampicin-resistant mutant derived from the wild-type isolateXooMAFF311018. Disease lesions were photographed at 25 d.p.i. Scale bar, 10 mm. (e) The lesions induced by infection with theXooT7174R were measured at 25 d.p.i. (f) The size of theXooT7174R population was determined at 5 d.p.i. Data shown inb,c,e,fare the means±s.d. for three individual experiments. Asterisks indicate significant differences between wild-type andXopPXoo-OX plants (Student’st-testPvalues,P<0.05). (g) Expression levels ofPBZ1andPAL1in wild-type (WT) andXopPXoo-OX cells after treatments with 100 μg ml−1PGN were analysed using quantitative RT–PCR. (h) Expression levels ofPBZ1andPAL1in WT andXopPXoo-OX cells after treatments with 2 μg ml−1chitin were analysed using quantitative RT–PCR. Data shown ing,hare the means±s.d. calculated using three biological replicates, where each biological replicate consists of two technical replicates. Asterisks indicate significant differences between WT andXopPXoo-OX cells (Student’st-testPvalues,P<0.05). Figure 1: XopP Xoo suppresses host immune responses. ( a ) Transgenic plants expressing XopP Xoo were more susceptible to the Xoo hrpX mutant. Disease lesions were photographed at 25 d.p.i. Scale bar, 10 mm. ( b ) The lesions induced by infection with the Xoo hrpX mutant were measured at 25 d.p.i. ( c ) The size of the Xoo hrpX mutant population in two independent XopP Xoo -OX transgenic lines was determined at 5 d.p.i. CFU, colony-forming unit. ( d ) Transgenic plants expressing XopP Xoo were more susceptible to Xoo T7174R, a spontaneous rifampicin-resistant mutant derived from the wild-type isolate Xoo MAFF311018. Disease lesions were photographed at 25 d.p.i. Scale bar, 10 mm. ( e ) The lesions induced by infection with the Xoo T7174R were measured at 25 d.p.i. ( f ) The size of the Xoo T7174R population was determined at 5 d.p.i. Data shown in b , c , e , f are the means±s.d. for three individual experiments. Asterisks indicate significant differences between wild-type and XopP Xoo -OX plants (Student’s t -test P values, P <0.05). ( g ) Expression levels of PBZ1 and PAL1 in wild-type (WT) and XopP Xoo -OX cells after treatments with 100 μg ml −1 PGN were analysed using quantitative RT–PCR. ( h ) Expression levels of PBZ1 and PAL1 in WT and XopP Xoo -OX cells after treatments with 2 μg ml −1 chitin were analysed using quantitative RT–PCR. Data shown in g , h are the means±s.d. calculated using three biological replicates, where each biological replicate consists of two technical replicates. Asterisks indicate significant differences between WT and XopP Xoo -OX cells (Student’s t -test P values, P <0.05). Full size image To analyse the PTI-inhibitory activity of XopP Xoo , we generated two suspension-cultured cell lines derived from callus lines independently transformed with the XopP Xoo -OX construct. The expression of XopP Xoo mRNA in rice cells was confirmed by semi-quantitative RT–PCR ( Supplementary Fig. 4 ). We treated these XopP Xoo -OX cells with a bacterial MAMP PGN. Quantitative RT–PCR indicated that the expression of two defence-related genes, Probenazole1 ( PBZ1 ) [30] and Phenylalanine ammonia-lyase1 ( PAL1 ) [31] , was significantly suppressed in the XopP Xoo -OX cells ( Fig. 1g ). In addition, we also treated these suspension-cultured cells with chitin, a fungal MAMP. The chitin-induced expression of PBZ1 and PAL1 was also reduced in the XopP Xoo -OX cell lines ( Fig. 1h ). These data indicate that XopP Xoo inhibits PTI induced by both PGN and chitin. However, it was noted that expression of XopP Xoo in rice cells did not influence chitin-induced activation of MAP kinases ( Supplementary Fig. 5 ). Identification of OsPUB44 as a host target for XopP Xoo To elucidate how XopP Xoo suppresses host immune responses, we screened host proteins capable of interacting with XopP Xoo by a yeast two-hybrid assay using a rice complementary DNA library prepared from chitin-treated rice suspension cells [32] . We isolated five positive clones as potential candidates for host targets of XopP Xoo from 8 × 10 5 cDNA clones. All five candidates corresponded to OsPUB44 (Os05g0439400) encoding a putative PUB E3 ubiquitin ligase with a U-box domain and a carboxy-terminal armadillo (ARM) repeat domain [7] . OsPUB44 belongs to the class III PUB family that includes CMPG1 and AtPUB22, AtPUB23 and AtPUB24, all known to be involved in immune responses [9] , [10] , [33] . The deduced OsPUB44 protein is 452 amino-acid residues in length. Full-length OsPUB44 interacted with XopP Xoo in yeast cells ( Fig. 2a ). We analysed the expression of OsPUB44 mRNA in response to PGN and chitin using wild-type rice suspension cells. The levels of OsPUB44 mRNA were markedly increased by both PGN and chitin treatments ( Fig. 2b ). The immunoblot treated with OsPUB44-specific antibody indicated that the levels of OsPUB44 protein were also increased with PGN and chitin treatments ( Fig. 2c ). 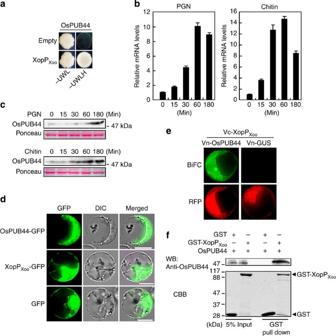Figure 2: XopPXoointeracts with OsPUB44. (a) Interaction between XopPXooand OsPUB44 in a yeast two-hybrid assay. The growth of yeast colonies on the plate (–ULWH) lacking uracil (U), leucine (L), tryptophan (W) and histidine (H) indicates a positive interaction. (b) Transcript levels ofOsPUB44mRNA in rice suspension-cultured cells after treatments with 100 μg ml−1PGN or 2 μg ml−1chitin were analysed using quantitative RT–PCR. Data are the means±s.d. for three individual experiments. (c)The protein levels of OsPUB44 in rice suspension-cultured cells after treatments with 100 μg ml−1PGN or 2 μg ml−1chitin were determined by treating an immunoblot with an OsPUB44-specific antibody. Molecular weight of protein: OsPUB44=48 kDa. (d) Subcellular localization of OsPUB44-GFP, XopPXoo-GFP and GFP in transiently transfected rice protoplasts. Fluorescence was observed 18 h after transformation. Scale bar, 10 μm. (e) Visualization of the interaction between XopPXooand OsPUB44 using a BiFC assay in transiently transfected rice protoplasts. Vn-XopPXooand Vc-OsPUB44 contain the N-terminal and C-terminal fragments, respectively, of Venus. The interaction between XopPXooand OsPUB44 was indicated by Venus fluorescence. Vn-GUS was used as a negative control. The fluorescence was observed 18 h after transformation. Scale bar, 10 μm. (f)In vitrointeraction between XopPXooand OsPUB44. OsPUB44 was incubated with GST or GST-XopPXooand then pulled down with glutathione-Sepharose 4B beads. OsPUB44 was detected by immunoblotting using an anti-OsPUB44 antibody. GST-XopPXoowas detected by Coomassie brilliant blue (CBB) staining. Molecular weights of proteins: OsPUB44=48 kDa, GST-XopPXoo=107 kDa, GST=28 kDa. Figure 2: XopP Xoo interacts with OsPUB44. ( a ) Interaction between XopP Xoo and OsPUB44 in a yeast two-hybrid assay. The growth of yeast colonies on the plate (–ULWH) lacking uracil (U), leucine (L), tryptophan (W) and histidine (H) indicates a positive interaction. ( b ) Transcript levels of OsPUB44 mRNA in rice suspension-cultured cells after treatments with 100 μg ml −1 PGN or 2 μg ml −1 chitin were analysed using quantitative RT–PCR. Data are the means±s.d. for three individual experiments. ( c )The protein levels of OsPUB44 in rice suspension-cultured cells after treatments with 100 μg ml −1 PGN or 2 μg ml −1 chitin were determined by treating an immunoblot with an OsPUB44-specific antibody. Molecular weight of protein: OsPUB44=48 kDa. ( d ) Subcellular localization of OsPUB44-GFP, XopP Xoo -GFP and GFP in transiently transfected rice protoplasts. Fluorescence was observed 18 h after transformation. Scale bar, 10 μm. ( e ) Visualization of the interaction between XopP Xoo and OsPUB44 using a BiFC assay in transiently transfected rice protoplasts. Vn-XopP Xoo and Vc-OsPUB44 contain the N-terminal and C-terminal fragments, respectively, of Venus. The interaction between XopP Xoo and OsPUB44 was indicated by Venus fluorescence. Vn-GUS was used as a negative control. The fluorescence was observed 18 h after transformation. Scale bar, 10 μm. ( f ) In vitro interaction between XopP Xoo and OsPUB44. OsPUB44 was incubated with GST or GST-XopP Xoo and then pulled down with glutathione-Sepharose 4B beads. OsPUB44 was detected by immunoblotting using an anti-OsPUB44 antibody. GST-XopP Xoo was detected by Coomassie brilliant blue (CBB) staining. Molecular weights of proteins: OsPUB44=48 kDa, GST-XopP Xoo =107 kDa, GST=28 kDa. Full size image To examine the subcellular localization of XopP Xoo and OsPUB44 in planta , green fluorescent protein (GFP) was fused to the C termini of XopP Xoo and OsPUB44, and constructs were expressed in rice protoplasts. Fluorescence for XopP Xoo -GFP and OsPUB44-GFP was detected in the entire region ( Fig. 2d ). Expression of these GFP-fused proteins was confirmed by immunoblot analysis ( Supplementary Fig. 6 ). In addition, the amino-terminal GFP fusions, GFP-XopP Xoo and GFP-OsPUB44, were also localized in the entire region ( Supplementary Fig. 7 ). We performed bimolecular fluorescence complementation (BiFC) to analyse the interaction between OsPUB44 and XopP Xoo in rice cells. OsPUB44 was tagged with the N-terminal domain (1–154 aa) of Venus (Vn-OsPUB44), and XopP Xoo was tagged with the C-terminal domain (155–238 aa) of Venus (Vc-XopP Xoo ). Co-expression of Vc-XopP Xoo with Vn-OsPUB44 in rice protoplasts resulted in fluorescence complementation in the entire region ( Fig. 2e ), suggesting the in vivo interaction of XopP Xoo with OsPUB44. In addition, an in vitro pull-down assay was used to confirm the interaction between OsPUB44 and XopP Xoo . We prepared OsPUB44 and glutathione S-transferase (GST)-fused XopP Xoo using a protein expression system in Escherichia coli . OsPUB44 was pulled down with GST-XopP Xoo , whereas GST alone did not interact with OsPUB44 ( Fig. 2f ). These data indicate that OsPUB44 directly interacts with XopP Xoo . OsPUB44 plays a role in PAMPs-triggered immunity To determine whether OsPUB44 is involved in PTI, we produced transgenic rice suspension cells carrying the OsPUB44 RNAi construct ( Supplementary Fig. 8 ). Both transcript and protein levels of OsPUB44 were significantly reduced in two independent OsPUB44 RNAi lines ( Fig. 3a,b ; Supplementary Fig. 9 ). PGN- and chitin-induced expressions of PBZ1 and PAL1 were significantly suppressed in both RNAi lines ( Fig. 3c,d ), whereas chitin-induced activation of MAP kinases was not altered in the OsPUB44 RNAi line ( Supplementary Fig. 10 ). These data coincided with the results of the XopP Xoo -OX lines. We also produced transgenic rice plants carrying the OsPUB44 RNAi construct ( Supplementary Fig. 11 ) and tested whether silencing of OsPUB44 affects resistance to the Xoo hrpX mutant using two independent RNAi plant lines. The O sPUB44 RNAi plants developed larger disease lesions than the wild type ( Fig. 3e ; Supplementary Fig. 12a ). The size of the bacterial population in the Xoo hrpX mutant in OsPUB44- RNAi leaves was significantly higher than in wild-type plants ( Fig. 3f ). We also analysed the disease resistance of the OsPUB44 RNAi plants to Xoo T7174R. Although we did not detect a significant difference in lesion lengths between the wild-type and the OsPUB44 RNAi plants ( Fig. 3g ; Supplementary Fig. 12b ), the amount of bacterial growth indicated that the OsPUB44 plants were more susceptible to Xoo T7174R as compared with wild-type plants ( Fig. 3h ). Thus, it is likely that OsPUB44 positively regulates PTI and Xoo resistance in rice. 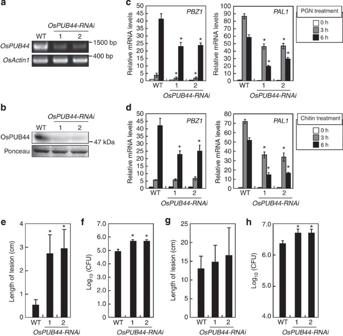Figure 3: OsPUB44 positively regulates PTI. (a) Transcript levels ofOsPUB44in theOsPUB44RNAi cells were analysed by RT–PCR. OsActin1 was used as a control. Molecular sizes of DNA fragments:OsPUB44=1,359 bp,OsActin1=387 bp. (b) The protein levels of OsPUB44 in theOsPUB44RNAi cells were determined by immunoblot analysis with the OsPUB44-specific antibody. Molecular weight of protein: OsPUB44=48 kDa. (c) Expression levels ofPBZ1andPAL1in wild-type andOsPUB44RNAi cells after treatments with 100 μg ml−1PGN were analysed using quantitative RT–PCR. (d) Expression levels ofPBZ1andPAL1in wild-type andOsPUB44RNAi cells after treatments with 2 μg ml−1chitin were analysed using quantitative RT–PCR. Data shown inc,dare the means±s.d. for three individual experiments. Asterisks indicate significant differences between WT andOsPUB44RNAi cells (Student’st-testPvalues,P<0.05). (e) Plants transformed with theOsPUB44RNAi construct were more susceptible to theXoo hrpXmutant. The lesions induced by infection with theXoo hrpXmutant were measured at 25 d.p.i. (f) The size of theXoo hrpXmutant population in theOsPUB44RNAi plants was determined at 5 d.p.i. CFU, colony-forming unit. (g) The disease lesions of the OsPUB44 RNAi plants induced by infection withXooT7174R were measured at 25 d.p.i. (h) The size of theXooT7174R population in theOsPUB44RNAi plants was determined at 5 d.p.i. Data shown ine–hare the means±s.d. calculated using three biological replicates, where each biological replicate consists of two technical replicates. Asterisks indicate significant differences between wild type and RNAi line 1, or RNAi line 2 (Student’st-testPvalues,P<0.05). Figure 3: OsPUB44 positively regulates PTI. ( a ) Transcript levels of OsPUB44 in the OsPUB44 RNAi cells were analysed by RT–PCR. OsActin1 was used as a control. Molecular sizes of DNA fragments: OsPUB44 =1,359 bp, OsActin1 =387 bp. ( b ) The protein levels of OsPUB44 in the OsPUB44 RNAi cells were determined by immunoblot analysis with the OsPUB44-specific antibody. Molecular weight of protein: OsPUB44=48 kDa. ( c ) Expression levels of PBZ1 and PAL1 in wild-type and OsPUB44 RNAi cells after treatments with 100 μg ml −1 PGN were analysed using quantitative RT–PCR. ( d ) Expression levels of PBZ1 and PAL1 in wild-type and OsPUB44 RNAi cells after treatments with 2 μg ml −1 chitin were analysed using quantitative RT–PCR. Data shown in c , d are the means±s.d. for three individual experiments. Asterisks indicate significant differences between WT and OsPUB44 RNAi cells (Student’s t -test P values, P <0.05). ( e ) Plants transformed with the OsPUB44 RNAi construct were more susceptible to the Xoo hrpX mutant. The lesions induced by infection with the Xoo hrpX mutant were measured at 25 d.p.i. ( f ) The size of the Xoo hrpX mutant population in the OsPUB44 RNAi plants was determined at 5 d.p.i. CFU, colony-forming unit. ( g ) The disease lesions of the OsPUB44 RNAi plants induced by infection with Xoo T7174R were measured at 25 d.p.i. ( h ) The size of the Xoo T7174R population in the OsPUB44 RNAi plants was determined at 5 d.p.i. Data shown in e – h are the means±s.d. calculated using three biological replicates, where each biological replicate consists of two technical replicates. Asterisks indicate significant differences between wild type and RNAi line 1, or RNAi line 2 (Student’s t -test P values, P <0.05). Full size image XopP Xoo inhibits the ubiquitin ligase activity of OsPUB44 To identify the PTI-inhibitory mechanism mediated by XopP Xoo , we analysed the domains of OsPUB44 that could interact with XopP Xoo using yeast two-hybrid analysis. As shown in Fig. 4a , we generated four constructs containing the U-box and/or ARM domain with or without a linker domain (103–203 aa) that were designated as OsPUB44 1–452 , OsPUB44 1–102 , OsPUB44 1–203 and OsPUB44 102–452 . XopP Xoo was shown to interact with OsPUB44 1–102 and OsPUB44 1–203 , but not with OsPUB44 102–452 ( Fig. 4b ). In addition, OsPUB44 1–203 interacted with XopP Xoo more strongly than OsPUB44 1–102 , which resulted from lower protein level of OsPUB44 1–102 in yeast ( Supplementary Fig. 13 ). 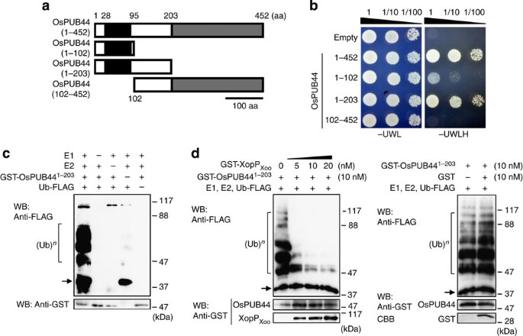Figure 4: XopPXooinhibits the ubiquitin E3 ligase activity of OsPUB44. (a) Schematic structures of full-length OsPUB441–452and three truncated OsPUB44 fragments, OsPUB441–102(1–102 aa), OsPUB441–203(1–203 aa) and OsPUB44102–452(102–452 aa). Black and grey boxes indicate the conserved U-box and ARM repeat domains, respectively. Numbers above the boxes indicate amino-acid residues. (b) Interaction of XopPXoowith OsPUB441–452, OsPUB441–102, OsPUB441–203and OsPUB44102–452in a yeast two-hybrid assay. (c)In vitroubiquitination assays of the OsPUB44 protein. The GST-OsPUB441–203protein was incubated with or without E1, E2 and ubiquitin (Ub)-FLAG. Ubiquitinated OsPUB441–203proteins were detected with an anti-FLAG antibody (upper panel). The presence of GST-OsPUB441–203protein was confirmed by immunoblotting using an anti-GST antibody (lower panel). Molecular weight of protein: GST-OsPUB441–203=48 kDa. Arrow indicates ubiquitin-loaded E2 proteins. Same results were obtained in more than three experiments. (d) The ubiquitin ligase activity of OsPUB44 was inhibited by XopPXoo. Anin vitroubiquitination assay of GST-OsPUB441–203was performed with or without GST-XopPXoo. Ubiquitinated OsPUB441–203was detected with an anti-FLAG antibody (upper panel). The presence of GST-OsPUB441–203and GST-XopPXooproteins was confirmed by immunoblotting using an anti-GST antibody (lower panel). The GST protein was detected by Coomassie brilliant blue staining. Molecular weights of proteins: GST-OsPUB441–203=48 kDa, GST-XopPXoo=107 kDa, GST=28 kDa. Arrow indicates ubiquitin-loaded E2 proteins. Same results were obtained in more than three experiments. Figure 4: XopP Xoo inhibits the ubiquitin E3 ligase activity of OsPUB44. ( a ) Schematic structures of full-length OsPUB44 1–452 and three truncated OsPUB44 fragments, OsPUB44 1–102 (1–102 aa), OsPUB44 1–203 (1–203 aa) and OsPUB44 102–452 (102–452 aa). Black and grey boxes indicate the conserved U-box and ARM repeat domains, respectively. Numbers above the boxes indicate amino-acid residues. ( b ) Interaction of XopP Xoo with OsPUB44 1–452 , OsPUB44 1–102 , OsPUB44 1–203 and OsPUB44 102–452 in a yeast two-hybrid assay. ( c ) In vitro ubiquitination assays of the OsPUB44 protein. The GST-OsPUB44 1–203 protein was incubated with or without E1, E2 and ubiquitin (Ub)-FLAG. Ubiquitinated OsPUB44 1–203 proteins were detected with an anti-FLAG antibody (upper panel). The presence of GST-OsPUB44 1–203 protein was confirmed by immunoblotting using an anti-GST antibody (lower panel). Molecular weight of protein: GST-OsPUB44 1–203 =48 kDa. Arrow indicates ubiquitin-loaded E2 proteins. Same results were obtained in more than three experiments. ( d ) The ubiquitin ligase activity of OsPUB44 was inhibited by XopP Xoo . An in vitro ubiquitination assay of GST-OsPUB44 1–203 was performed with or without GST-XopP Xoo . Ubiquitinated OsPUB44 1–203 was detected with an anti-FLAG antibody (upper panel). The presence of GST-OsPUB44 1–203 and GST-XopP Xoo proteins was confirmed by immunoblotting using an anti-GST antibody (lower panel). The GST protein was detected by Coomassie brilliant blue staining. Molecular weights of proteins: GST-OsPUB44 1–203 =48 kDa, GST-XopP Xoo =107 kDa, GST=28 kDa. Arrow indicates ubiquitin-loaded E2 proteins. Same results were obtained in more than three experiments. Full size image To address whether OsPUB44 possesses the E3 ubiquitin ligase activity, OsPUB44 1–203 was fused to GST and expressed in E. coli . The GST-fused OsPUB44 1–203 was incubated with E1 enzyme, E2 enzyme (UbcH6) and Flag-tagged ubiquitin. The ubiquitinated proteins were detected by immunoblot analysis using anti-FLAG antibody. As shown in Fig. 4c , OsPUB44 1–203 had significant ubiquitin ligase activity in the presence of all the essential reaction components. We also analysed the ubiquitin ligase activity of full-length OsPUB44 1–452 . Full-length OsPUB44 1–452 had significant ubiquitin ligase activity, although much less activity than that of OsPUB44 1–203 ( Supplementary Fig. 14 ). The interaction of XopP Xoo with the U-box domain of OsPUB44 raised a possibility that XopP Xoo may inhibit the ubiquitin ligase activity. Therefore, we carried out an in vitro ubiquitin ligase assay of the U-box domain in the presence of XopP Xoo . The ubiquitin ligase activity was significantly reduced by the addition of GST-XopP Xoo in a dose dependent manner ( Fig. 4d ), whereas GST did not affect the activity. These data strongly suggest that the OsPUB44 ubiquitin ligase activity is suppressed by XopP Xoo by direct binding. The ubiquitin E3 ligases are known to regulate their own protein levels by autocatalytic ubiquitination-mediated protein turnover. In fact, the inactive mutants of AtPUB22 were found to be stable and could accumulate to high levels in the cells [34] . Therefore, if XopP Xoo inhibits OsPUB44 activity in vivo , the inactivated OsPUB44 should accumulate in the XopP Xoo -OX cells. The protein levels of OsPUB44 were compared between wild-type and the XopP Xoo -OX cells after treatments with PGN or chitin. We found that the OsPUB44 proteins accumulated in XopP Xoo -OX cells to higher levels than in wild type ( Fig. 5a ). The protein levels of OsPUB44 in the XopP Xoo -OX cells were more than 15-fold higher as compared with those in wild type at 30 min after treatments with PGN and chitin. These data support the idea that XopP Xoo interacts with the U-box domain in vivo and inhibits ubiquitin ligase activity, resulting in stabilization of OsPUB44 in the cells. 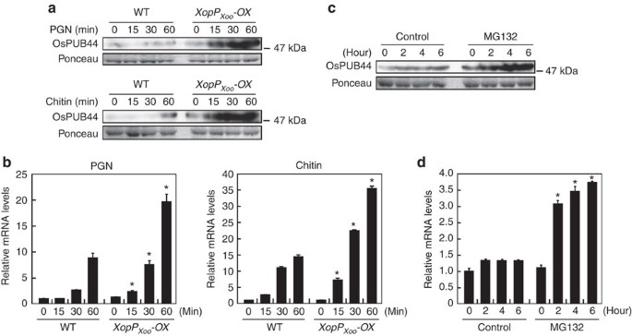Figure 5: OsPUB44 is accumulated in the presence of XopPXoo. (a) OsPUB44 was stabilized in the presence of XopPXoo. The protein levels of OsPUB44 in wild-type (WT) andXopPXoo-OX cells after treatments with 100 μg ml−1PGN or 2 μg ml−1chitin were determined by immunoblot analysis with the OsPUB44-specific antibody. Molecular weight of protein: OsPUB44=48 kDa. (b) Transcript levels ofOsPUB44mRNA in WT andXopPXoo-OX cells after treatment with 100 μg ml−1PGN or 2 μg ml−1chitin were analysed using quantitative RT–PCR. Data are the means±s.d. for three individual experiments. Asterisks indicate significant differences between WT andXopPXoo-OX cells (Student’st-testPvalues,P<0.05). (c) The protein levels of OsPUB44 in rice cells after treatment with the proteasomal inhibitor MG132 (30 μM) or an equivalent volume of dimethylsulphoxide (DMSO; control) were determined by immunoblot analysis with the OsPUB44-specific antibody. Molecular weight of protein: OsPUB44=48 kDa. (d) Transcript levels ofOsPUB44mRNA in rice cells after treatment with the proteasomal inhibitor MG132 (30 μM) or an equivalent volume of DMSO (control) were analysed using quantitative RT–PCR. Data are the means±s.d. for three individual experiments. Asterisks indicate significant differences between control and MG132-treated cells (Student’st-testPvalues,P<0.05). Figure 5: OsPUB44 is accumulated in the presence of XopP Xoo . ( a ) OsPUB44 was stabilized in the presence of XopP Xoo . The protein levels of OsPUB44 in wild-type (WT) and XopP Xoo -OX cells after treatments with 100 μg ml −1 PGN or 2 μg ml −1 chitin were determined by immunoblot analysis with the OsPUB44-specific antibody. Molecular weight of protein: OsPUB44=48 kDa. ( b ) Transcript levels of OsPUB44 mRNA in WT and XopP Xoo -OX cells after treatment with 100 μg ml −1 PGN or 2 μg ml −1 chitin were analysed using quantitative RT–PCR. Data are the means±s.d. for three individual experiments. Asterisks indicate significant differences between WT and XopP Xoo -OX cells (Student’s t -test P values, P <0.05). ( c ) The protein levels of OsPUB44 in rice cells after treatment with the proteasomal inhibitor MG132 (30 μM) or an equivalent volume of dimethylsulphoxide (DMSO; control) were determined by immunoblot analysis with the OsPUB44-specific antibody. Molecular weight of protein: OsPUB44=48 kDa. ( d ) Transcript levels of OsPUB44 mRNA in rice cells after treatment with the proteasomal inhibitor MG132 (30 μM) or an equivalent volume of DMSO (control) were analysed using quantitative RT–PCR. Data are the means±s.d. for three individual experiments. Asterisks indicate significant differences between control and MG132-treated cells (Student’s t -test P values, P <0.05). Full size image The PGN- and chitin-induced expression levels of OsPUB44 mRNA were slightly but significantly higher in the XopP Xoo -OX cells as compared with wild type ( Fig. 5b ), although the increased levels of OsPUB44 mRNA in the XopP Xoo -OX cells was much lower as compared with the increased levels of OsPUB44 proteins. It is possible that the slight increase in mRNA levels may be caused by the inhibition of OsPUB44 turnover. To test this possibility, rice cells were treated with a proteasome inhibitor MG132. Treatment with MG132 induced accumulation of the OsPUB44 protein ( Fig. 5c ), and also increased the transcript levels ( Fig. 5d ). These data suggest that inhibition of protein turnover of the OsPUB44 protein may enhance its transcription or stability of the transcript. OsPUB44 possesses a unique U-box domain A phylogenetic analysis of the U-box family indicated that the U-box domain of OsPUB44 is highly homologous to those of OsPUB45 (Os02g0540700) and OsPUB46 (Os04g0418500; Supplementary Fig. 15 ). We examined the interaction of XopP Xoo with OsPUB45 and OsPUB46 ( Fig. 6a ); however, no interactions were detected, although these proteins were expressed in yeast ( Supplementary Fig. 16 ). Therefore, we compared the amino-acid sequences of the OsPUB44 U-box domain with those of OsPUB45 and OsPUB46, and Arabidopsis orthologues AtPUB27, AtPUB28 and AtPUB29. Eight amino-acid residues within the U-box domain of OsPUB44 varied from the corresponding residues of the closely related PUB proteins including OsPUB45 and OsPUB46 ( Fig. 6b ), suggesting that these eight amino-acid residues may determine the specificity of interaction with XopP Xoo . We produced OsPUB44 U-box mutants in which each of the OsPUB44-specific residues was substituted with the corresponding residues in OsPUB45 and OsPUB46. The interaction between XopP Xoo and the OsPUB44 1–203 mutants was analysed by the yeast two-hybrid method. We found that XopP Xoo did not interact with two mutants, OsPUB44 1–203, L86T and OsPUB44 1–203, H94W ( Fig. 6c ). Although OsPUB44 1–203, P48C also did not interact with XopP Xoo , this failure was caused by undetectable expression of OsPUB44 1–203, P48C in yeast ( Supplementary Fig. 16 ). To further examine whether L86 and H94 contribute to the interaction, we mutated two amino-acid residues (T133 and W141) of OsPUB45 with two residues corresponding to L86 and H94 of OsPUB44, and generated OsPUB45 1–234, T133L, W141H . The new construct, OsPUB45 1–234, T133L, W141H interacted with XopP Xoo ( Fig. 6d ), demonstrating that leucine and histidine corresponding to L86 and H94 of OsPUB44 are essential residues for interaction with XopP Xoo . 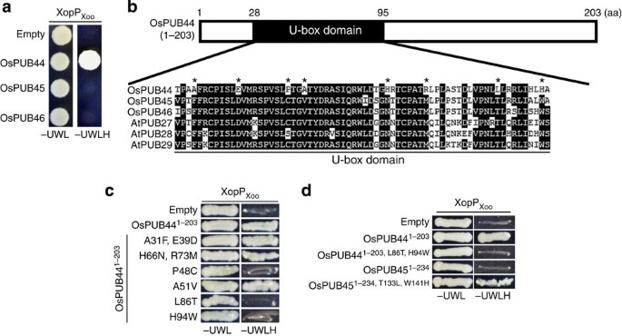Figure 6: OsPUB44 possesses a unique U-box domain. (a) Interaction of XopPXoowith OsPUB44, OsPUB45 and OsPUB46 in a yeast two-hybrid assay. (b) Eight amino-acid residues within the U-box domain of OsPUB44 are different from those of OsPUB44 homologues andArabidopsisorthologues. A comparison of the amino-acid sequence of the U-box domain of OsPUB44 with those of OsPUB45, OsPUB46, AtPUB27, AtPUB28 and AtPUB29 was performed using ClustalW2 software. The conserved amino-acid residues are shaded. Asterisks indicate the eight amino-acid residues specific for OsPUB44. (c) Interaction of XopPXoowith the substituted OsPUB441–203proteins in a yeast two-hybrid assay. (d) Interaction of XopPXoowith OsPUB451–234, T133L, W141Hin a yeast two-hybrid assay. Figure 6: OsPUB44 possesses a unique U-box domain. ( a ) Interaction of XopP Xoo with OsPUB44, OsPUB45 and OsPUB46 in a yeast two-hybrid assay. ( b ) Eight amino-acid residues within the U-box domain of OsPUB44 are different from those of OsPUB44 homologues and Arabidopsis orthologues. A comparison of the amino-acid sequence of the U-box domain of OsPUB44 with those of OsPUB45, OsPUB46, AtPUB27, AtPUB28 and AtPUB29 was performed using ClustalW2 software. The conserved amino-acid residues are shaded. Asterisks indicate the eight amino-acid residues specific for OsPUB44. ( c ) Interaction of XopP Xoo with the substituted OsPUB44 1–203 proteins in a yeast two-hybrid assay. ( d ) Interaction of XopP Xoo with OsPUB45 1–234, T133L, W141H in a yeast two-hybrid assay. Full size image We investigated whether the U-box proteins containing these two OsPUB44-specific residues generally exist in the plant kingdom. A database search did not find any PUB proteins with two residues corresponding to L86 and H94 of OsPUB44, except for OsPUB44. XopP Xoo targets the unique U-box domain of OsPUB44 Because OsPUB45 did not interact with XopP Xoo , we hypothesized that XopP Xoo could not inhibit the ubiquitin ligase activity of OsPUB45. The U-box domain of OsPUB45 had ubiquitin ligase activity in vitr o ( Fig. 7a ). However, the ligase activity of OsPUB45 was not suppressed in the presence of XopP Xoo , whereas the same amount of XopP Xoo inhibited the OsPUB44 activity ( Fig. 7b ). To investigate whether the two amino-acid residues (L86 and H94) responsible for interaction with XopP Xoo affect the inhibition of the OsPUB44 ligase activity by XopP Xoo , we prepared the recombinant OsPUB44 U-box protein with L86T and H94W in E. coli . The OsPUB44 1–203, L86T, H94W protein possessed E3 ligase activity that was not inhibited by XopP Xoo ( Fig. 7c ). In contrast, OsPUB45 U-box protein with T133L and W141H was inhibited by XopP Xoo ( Fig. 7d ). These data indicated that leucine and histidine corresponding to L86 and H94 of OsPUB44 are required for inhibition of the ligase activities by XopP Xoo . 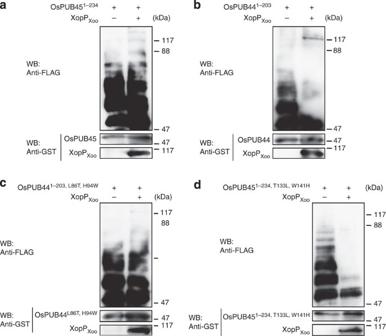Figure 7: XopPXoodoes not inhibit the ubiquitin E3 ligase activity of OsPUB45. The same amounts (10 nM) of GST-OsPUB451–234(a), GST-OsPUB441–203(b), OsPUB441–203, L86T, H94W(c) and OsPUB451–234, T133L, W141H(d) were incubated in a reaction mixture containing E1, E2 and ubiquitin (Ub)-FLAG with or without GST-XopPXoo(10 nM). Ubiquitinated proteins were detected with an anti-FLAG antibody (upper panels). The presence of GST-OsPUB441–203, GST-OsPUB451–234, GST-OsPUB441–203, L86T, H94W, OsPUB451–234, T133L, W141Hand GST-XopPXoowas confirmed by immunoblot analysis using anti-GST antibody (lower panels). Molecular weights of proteins: GST-OsPUB441–203=48 kDa, GST-OsPUB451–234=52 kDa, GST-XopPXoo=107 kDa. Similar results were obtained in more than three experiments. Figure 7: XopP Xoo does not inhibit the ubiquitin E3 ligase activity of OsPUB45. The same amounts (10 nM) of GST-OsPUB45 1–234 ( a ), GST-OsPUB44 1–203 ( b ), OsPUB44 1–203, L86T, H94W ( c ) and OsPUB45 1–234, T133L, W141H ( d ) were incubated in a reaction mixture containing E1, E2 and ubiquitin (Ub)-FLAG with or without GST-XopP Xoo (10 nM). Ubiquitinated proteins were detected with an anti-FLAG antibody (upper panels). The presence of GST-OsPUB44 1–203 , GST-OsPUB45 1–234 , GST-OsPUB44 1–203, L86T, H94W , OsPUB45 1–234, T133L, W141H and GST-XopP Xoo was confirmed by immunoblot analysis using anti-GST antibody (lower panels). Molecular weights of proteins: GST-OsPUB44 1–203 =48 kDa, GST-OsPUB45 1–234 =52 kDa, GST-XopP Xoo =107 kDa. Similar results were obtained in more than three experiments. Full size image U-box proteins are implicated in immunity and most function as negative regulators [10] , [11] , [13] . To date, only one U-box protein, CMPG1, has been identified as a positive immune regulator. CMPG1, originally identified as a gene rapidly induced after Cladosporum fulvum Avr9 elicitation in Cf-9 tobacco cells [35] , positively regulates cell death and disease resistance in several types of plant–microbe interactions [9] . In this study, we found that silencing OsPUB44 resulted in reduced expression of PGN- and chitin-induced defence genes and suppressed resistance to Xoo . These data strongly suggest that OsPUB44 is another positive regulator of immune responses. Since OsPUB44 and CMPG1 positively regulate immune responses, these proteins are likely important targets for pathogens to suppress host defence. CMPG1 is known to be targeted by P. infestans effector AVR3a [15] , [16] . AVR3a interacts with and stabilizes CMPG1, resulting in the inhibition of CMPG1. Nevertheless, how AVR3a stabilizes CMPG1 in plant cells and why CMPG1 function is lost by the stabilization remain to be identified. In this study, we discovered that XopP Xoo directly interacts with the U-box domain of OsPUB44, thereby reducing the E3 ligase activity. As found in the interaction between CMPG1 and AVR3a, the expression of XopP Xoo in host cells also stabilizes OsPUB44. The phenomenon may be explained by the hypothesis that XopP Xoo inhibits autocatalytic ubiquitination-mediated turnover of OsPUB44. This possibility is also supported by the observation that MG132-mediated inhibition of 26S proteasomes stabilized OsPUB44. These results indicate that stabilization of OsPUB44 occurs by inactivation of ligase activity. Although many pathogen effectors are known to target host proteins involved in the ubiquitin-proteasome pathway [8] , [14] , [15] , [16] , this is the first case documenting that pathogen effectors interact with the E3 ligase domain and modulate its activity. Other U-box proteins involved in immunity function as negative regulators. For example, Arabidopsis AtPUB12 and AtPUB13 ubiquitinate FLS2, a flagellin receptor, and then FLS2 is degraded in the proteasome pathway [11] , leading to attenuation of immune signalling. Arabidopsis AtPUB22, AtPUB23 and AtPUB24 redundantly and negatively regulate PTI [10] . In addition, AtPUB22 and AtPUB23 also function as negative regulators in the water-stress response [36] . Recently, Exo70B2, a component of the exocytic machinery, was identified as a substrate for AtPUB22 (ref. 34 ). AtPUB22 is proposed to control PTI by degradation of Exo70B2. Although a limited number of the U-box E3 ligases function as positive regulators, there are several RING-finger-type E3 ligases that positively regulate immune responses [8] . Recently, Park et al. [14] reported that M. oryzae effector AvrPiz-t targets rice RING finger-type E3 ubiqutin ligase APIP6, a positive regulator for PTI. Interestingly, APIP6 ubiquitinates AvrPiz-t in vitro . In fact, when AvrPiz-t and APIP6 are ectopically co-expressed in tobacco cells, AvrPiz-t is degraded in the presence of APIP6. In addition, the E3 ligase activity of APIP6 is reduced in the presence of AvrPiz-t; however, the molecular details of how AvrPiz-t reduces the ligase activity of APIP6 remain to be determined. In this study, we found that two amino-acid residues in the OsPUB44 U-box domain are responsible for interaction with XopP Xoo . Among 78 U-box proteins in rice, only OsPUB44 contains two unusual amino-acid residues. Although Arabidopsis contains 63 U-box proteins, there are no OsPUB44-type U-box proteins encoded in the Arabidopsis genome. How these unusual U-box proteins evolved is an intriguing question. Another important question is why XopP Xoo targets the unusual U-box domain. If XopP Xoo could interact with typical U-box domains, many U-box proteins would be influenced by XopP Xoo , which is an unsuitable condition for pathogen proliferation. For example, as mentioned above, AtPUB12, AtPUB13, AtPUB22, AtPUB23 and AtPUB24 negatively regulate immunity in Arabidopsis [10] , [11] . If XopP Xoo interacted with these negative regulators and inhibited their functions, enhanced immune responses would result. If XopP Xoo targeted the U-box proteins that play essential roles in host physiological processes, XopP Xoo would damage the host cells. Thus, it is likely that pathogen effectors require a high degree of specificity for interaction with host targets. Although XopP Xoo is classified into the XopP family, XopP Xoo has only 40% identity with the XopP homologue of X. campestris pv. campestris [18] . Therefore, Xcc XopP may possibly target other factors involved in immunity. The biochemical function of XopP Xoo cannot be predicted due to the lack of any known domains. Therefore, it is unclear whether the E3 ligase activity of OsPUB44 is inhibited by an enzymatic reaction of XopP Xoo or a physical interaction with XopP Xoo . Another possibility is that XopP Xoo may inhibit an interaction between OsPUB44 and E2 enzyme by competing for the binding site with E2 enzyme. Although we tested this hypothesis, the data were inconclusive from the in vitro interaction experiment. In some cases, the enzymatic properties of pathogen effectors have been discovered by determining the tertiary structures of effector proteins [37] . Crystal structures of XopP Xoo and/or OsPUB44 will help to reveal how XopP Xoo inhibits OsPUB44 activity at the molecular level. In Arabidopsis , AtPUB12 and AtPUB13 ubiquitinate FLS2, the extracellular leucine-rich repeats-containing receptor-like kinase [11] . Thus, it is possible that OsPUB44 may be associated with OsCERK1, a rice extracellular LysM domain-containing receptor-like kinase responsible for recognizing chitin and PGN. However, chitin-induced activation of MAP kinases was not altered in OsPUB44 RNAi and XopP Xoo -OX cells, suggesting that OsPUB44 as well as XopP Xoo may not regulate the protein level and the activity of OsCERK1. Recently, we identified rice receptor-like cytoplasmic kinase OsRLCK185 as a target for X. oryzae effector XopY Xoo and found that OsRLCK185 transmits the immune signal from OsCERK1 to the downstream MAP kinase cascade [19] . Since MAP kinase activation was not altered in the OsPUB44 RNAi cells, it is likely that OsPUB44 functions in a different pathway than OsRLCK185 or downstream of the MAPK cascade. Identification of the host proteins ubiquitinated by OsPUB44 will be a key factor in understanding how OsPUB44 regulates PAMPs-triggered immunity. Plasmid constructs Full-length cDNAs for OsPUB44 (Os05g0439400), OsPUB45 (Os02g0540700) and OsPUB46 (Os04g0418500) were amplified by PCR from cDNA pools prepared from leaves of rice cultivars Nipponbare or Kinmaze (primers are described in Supplementary Table 1 ). The coding region of XopP Xoo was amplified from genomic DNA prepared from X. oryzae pv. oryzae . Forward and reverse primers were designed on the basis of sequence information in the Rice Annotation Project Database ( http://rapdb.dna.affrc.go.jp/ ) or the Xanthomonas oryzae pv. oryzae Genome Database ( http://microbe.dna.affrc.go.jp/Xanthomonas/ ). The coding region of each gene was amplified by PCR and ligated into the pENTR/D-TOPO cloning vector (Invitrogen). To produce XopP Xoo -OX cells and plants, the XopP Xoo coding region was introduced into the p2K1 vector to control expression with the maize ubiquitin 1 promoter [38] . For RNAi vectors, a 514-bp (base pair) fragment of OsPUB44 was amplified, combined by PCR and cloned into pENTR/D-TOPO ( Supplementary Fig. 8 ). The 514-bp fragment was subcloned into the pANDA vector in the inverse orientation by one LR clonase reaction [39] . Point mutations of OsPUB44 were generated by PCR using primers designed to substitute the corresponding amino acids (primers are described in Supplementary Table 1 ). OsPUB44 A31F, E39D , OsPUB44 H66N, R73M , OsPUB44 P48C , OsPUB44 A51V , OsPUB44 L86T and OsPUB44 H94W were made by replacing Ala-31and Glu-39, His-66 and Arg-73, Pro-48, Ala-51, Leu-86 and His-94 in OsPUB44 with Phe and Glu, Asn and Met, Cys, Val, Thr and Trp, respectively. OsPUB45 T133L, W141H was made by replacing Thr-133 and Trp-141 in OsPUB45 with Leu and His, respectively. OsPUB44, OsPUB44 1–102 , OsPUB44 1–203 , OsPUB44 102–452 , OsPUB44 C34A , OsPUB44 V45I , OsPUB44 A31F, E39D , OsPUB44 H66N, R73M , OsPUB44 P48C , OsPUB44 A51V , OsPUB44 L86T , OsPUB44 H94W , OsPUB45, OsPUB45 T133L, W141H , OsPUB46 and XopP Xoo clones were transferred by the Gateway system using an LR clonase reaction into pBTM116-GW and pVP16-GW for the yeast two-hybrid assays [40] , into p35S-GFP-GW for subcellular localization assays, into p35S-Vn-GW and p35S-Vc-GW for the BiFC assay and into the p2K-GW binary vector to produce transgenic plants expressing trans genes under the control of the maize ubiquitin promoter [19] . Rice transformation Calli generated from embryos of rice cultivars Nipponbare or Kinmaze , which were used for XopP Xoo -OX or OsPUB44 RNAi, respectively, were transformed by infection of Agrobacterium tumefaciens EHA101 carrying corresponding constructs as described [41] . The transformed calli were selected by resistance to hygromycin and used for generation of T 0 plants. Suspension-cultured cells were also prepared from transformed calli or from calli generated from T 0 plant seeds. Yeast two-hybrid assays A yeast two-hybrid library was prepared using total RNA extracted from rice suspension cells that had been treated with chitin [32] . To construct the bait vector, the coding region of XopP Xoo was cloned into pBTM116. Screening was performed on synthetic complete (SC) medium lacking histidine. Combinations of the bait and prey vectors were introduced into cells of Saccharomyces cerevisiae L40 ( MATatrp1 leu2 his3 LYS2::lexA-HIS3 URA3::lexA-lacZ ). Transformants were selected on minimal medium lacking tryptophan and leucine. The two-hybrid interaction was analysed based on the histidine requirement for yeast growth as described previously [32] , [40] . PAMP treatment Rice suspension-cultured cells were subcultured for 3 days in fresh medium, divided into 12-well plates (150 mg cells, 2 ml fresh medium per well) and treated with 2 μg ml −1 hexa- N -acetylchitohexaose (Seikagaku Biobusiness) or 100 μg ml −1 PGN from Bacillus subtilis (Sigma). RNA isolation and RT–PCR analysis Total RNA was isolated from rice suspension-cultured cells using TRIzol reagent (Invitrogen) and then treated with RNase-free DNase I (Roche). First-strand cDNA was synthesized from 1 μg total RNA with an oligo-dT primer and ReverTra Ace (Toyobo). Expression levels were quantified by qRT–PCR using SYBR Green master mix (Applied Biosystems) in a Step-One Plus Real-Time PCR system (Applied Biosystems), and normalized against a ubiquitin reference gene. Three biological replicates were used for each experiment, and two quantitative iterations were performed for each biological replicate. Protein extraction and immunoblotting Total proteins were extracted in a buffer including 100 mM Tris–HCl, pH 7.5, 20% (v/v) glycerine and protease inhibitor cocktail (Roche) and analysed by protein immunoblotting with anti-OsPUB44 antibody (1:2,000 dilution), anti-GFP antibody (ab6556; Abcam, 1:2,000 dilution) or anti-pMAPK (4370; Cell Signaling, 1:2,000 dilution). Polyclonal antibody (prepared by MBL) for OsPUB44 was raised in rabbits using a polypeptide fragment (aa 330–452) from OsPUB44 as the antigen. The uncropped immunoblots are shown in Supplementary Fig. 17 ). Transient assays using rice protoplasts Protoplasts were isolated from cultured rice cells by digestion of cell wall with Cellulase RS (Yakult) and Macerozyme R-10 (Yakult) as previously described [42] . Plasmid transformations were performed using the polyethylene glycol method [43] . Aliquots (100 μl) of protoplasts prepared from suspension-cultured cells (2.5 × 10 6 cells ml −1 ) were transformed by mixing with 5 μg plasmid DNA. For localization analysis and BiFC assays, transfected protoplasts were observed using confocal microscopy (BZ-9000, Keyence, Japan). In vitro ubiquitination assays The OsPUB44 1–203 , OsPUB45 1–234 , OsPUB44 1–203, L86T, H94W , OsPUB45 1–234, L133T, H141W and XopP Xoo fragments were subcloned into a pCold GST vector [44] . These proteins were expressed as fusion proteins having a GST tag using a Cold-Shock Bacterial Expression System (Takara Bio) following the supplier’s instructions. Each protein was purified using glutathione-Sepharose 4B (GE Healthcare). Ubiquitination assays were performed as described previously [10] with minor modification. Protein samples (500 ng) of purified GST-OsPUB44 1–203 , OsPUB45 1–234 , and OsPUB44 1–203, L86T, H94W , OsPUB45 1–234, L133T, H141W and 0–20 nM purified GST-XopP Xoo were incubated in 30 μl reaction buffer containing 50 mM Tris–HCl, pH 7.5, 5 mM MgCl 2 , 4 mM ATP, 2 mM dithiothreitol (DTT), 30 ng yeast E1 (Wako), 200 ng UbcH6 for E2 (Wako) and 5 μg FLAG-ubiquitin (Sigma-Aldrich). Reactions were stopped by adding sample buffer (125 mM Tris–HCl, pH 6.8, 20% (v/v) glycerine, 4% (w/v) SDS and 0.4 M DTT) and were then analysed by SDS–PAGE followed by protein immunoblot analysis using an anti-FLAG antibody (F3165; Sigma-Aldrich (1:2,000 dilution)) or an anti-GST antibody (04435-26; Nacalai Tesque (1:5,000 dilution)). In vitro pull-down assays The full-length OsPUB44 protein was purified by removing the GST tag through digestion with Turbo 3C protease (Nacalai Tesque). OsPUB44 was incubated with GST-XopP Xoo or GST at 30 °C for 15 min in a reaction buffer (50 mM Tris–HCl, pH 7.5, 5 mM MgCl 2 , 4 mM ATP and 2 mM DTT). Glutathione-Sepharose 4B beads were added and the mixture was incubated at 4 °C for 15 min, and then washed five times with a washing buffer (50 mM Tris–HCl, pH 7.5, 300 mM NaCl and 1 mM DTT). After the final wash, bound proteins were eluted with SDS sample buffer and subjected to protein immunoblot analysis. Pathology assays X. oryzae pv . oryzae (Xoo) strains were cultured on NBY plates containing either rifampicin (20 μg ml −1 ) for Xoo T7174R, a spontaneous rifampicin-resistant mutant derived from wild-type MAFF311018, or rifampicin/kanamycin (25 μg ml −1 ) for the Xoo hrpX strain for 3 days at 28 °C. Fully expanded rice leaves were inoculated by clipping leaf tips with scissors that had been immersed in bacterial suspensions (OD 600 =0.3) [45] . Symptoms were scored by measuring lesion lengths 25 days post inoculation (d.p.i.). Bacterial growth in planta was measured as reported previously [18] . The inoculated rice leaves (1 cm long) were collected at 5 d.p.i. Leaves were ground in and diluted with sterile water and then plated on the peptone-sucrose medium containing rifampicin or rifampicin and kanamycin for direct colony counts. How to cite this article: Ishikawa, K. et al. Bacterial effector modulation of host E3 ligase activity suppresses PAMP-triggered immunity in rice. Nat. Commun. 5:5430 doi: 10.1038/ncomms6430 (2014).